FLOWERING LOCUS C in monocots and the tandem origin of angiosperm-specific MADS-box genes MADS-domain transcription factors have been shown to act as key repressors or activators of the transition to flowering and as master regulators of reproductive organ identities. Despite their important roles in plant development, the origin of several MADS-box subfamilies has remained enigmatic so far. Here we demonstrate, through a combination of genome synteny and phylogenetic reconstructions, the origin of three major, apparently angiosperm-specific MADS-box gene clades: FLOWERING LOCUS C- ( FLC- ), SQUAMOSA- ( SQUA- ) and SEPALLATA- ( SEP- ) -like genes. We find that these lineages derive from a single ancestral tandem duplication in a common ancestor of extant seed plants. Contrary to common belief, we show that FLC- like genes are present in cereals where they can also act as floral repressors responsive to prolonged cold or vernalization. This opens a new perspective on the translation of findings from Arabidopsis to cereal crops, in which vernalization was originally described. Flowering plants have evolved an enormous complexity and diversity in the developmental transition from vegetative to reproductive growth. Environmental and internal cues are integrated in a quantitative flowering response that varies between species and even between ecotypes [1] . Plants growing in temperate climates use photoperiod or day-length, in addition to vernalization or low temperatures to sense the passing of winter into optimal reproductive environmental conditions [2] . The elaboration of reproductive development in flowering plants is associated with the origin and diversification of developmental control genes, most prominently members of the MADS-box transcription factor family. The origin of several subfamilies of MADS-box genes with crucial roles in the floral transition remains shrouded in mystery, in that they appear to be present in just flowering plants or in specific lineages of flowering plants. One lineage of MADS-box genes with a highly enigmatic origin is the clade of FLOWERING LOCUS C ( FLC ) genes. In the model plant Arabidopsis thaliana , FLC is a central repressor of the floral transition [3] , where it inhibits flowering by directly repressing the activity of central flowering promoters, namely SUPPRESSOR OF OVEREXPRESSION OF CONSTANS ( SOC1 ), FLOWERING LOCUS D ( FD ) and FLOWERING LOCUS T ( FT ) [1] , [2] , [3] , [4] , [5] . Vernalization alleviates this repression by negatively regulating FLC expression through epigenetic modifications of the chromatin structure at the FLC locus [2] , [4] . FLC has five closely related paralogs in the Arabidopsis thaliana genome, some of which also act as floral repressors [6] , [7] , [8] . These paralogs arose in evolution through sequential tandem and genome duplications within the order Brassicales [9] , [10] . Tandem duplications of FLC -like genes are not uncommon, as they have also been reported in other Arabidopsis species [10] . Outside of Brassicales FLC -like genes have been identified in more distantly related core eudicot species. For instance in sugar beet ( Beta vulgaris ), a crop with a strong vernalization requirement, FLC expression also responds to vernalization [11] . FLC homologues, however, have not been identified outside the core eudicots and the phylogenetic position of this subfamily in the larger MADS-box gene phylogeny, and therefore its evolutionary origin, is uncertain. Historically, vernalization has been extensively studied in temperate monocot crops, like winter varieties of wheat and barley [12] . To significantly accelerate flowering and subsequent seed set, winter cereals require a sufficiently long period of cold. In contrast to Arabidopsis, however, their vernalization response involves other members of the MADS-box gene family, as well as other genes [12] , [13] , [14] . Therefore, it has previously been suggested that the vernalization response in temperate cereals and eudicots may have evolved independently [13] , [14] , [15] . FLC -like genes are not the only subfamily of MADS-box genes with an enigmatic origin. While members of the SQUAMOSA ( SQUA ) and SEPALLATA ( SEP ) subfamilies have been identified in all major flowering plant lineages, no gymnosperm representatives have so far been found despite the availability of extensive transcriptome investigations and targeted cloning efforts [16] , [17] . In angiosperms, rounds of polyploidization (whole-genome duplications) probably generated many of the observed gene duplications in the SQUA and SEP subfamilies [18] , [19] , [20] , [21] . Members of the SQUA subfamily are generally positive regulators of the floral transition as they control the formation of inflorescence and floral meristems [22] . SEP genes act as key regulators of floral organ specification, and in a partially redundant manner with SQUA- like genes in floral meristem specification [23] , [24] . Clarifying the origin of SEP , SQUA and FLC subfamilies can greatly contribute to our understanding of the evolution of flowering plants. In this study, we combined genomic synteny-based approaches and phylogeny reconstruction to understand the evolutionary history of these MADS-box gene subfamilies. This allowed us to identify FLC orthologs in monocots. Similar to Arabidopsis FLC , the expression of Brachypodium FLC -like genes is responsive to a prolonged cold period. The tandem arrangement of the FLC , SEP and SQUA subfamilies suggests an origin of these subfamilies by an ancient tandem duplication before the origin of extant flowering plants, followed by segmental duplications linked to rounds of polyploidization. Our results close an important gap in our understanding on the origin of developmental key regulatory genes in flowering plants. Conserved SEP3-FLC and SEP1-SQUA tandems in core eudicots The conservation of gene order between species and between duplicated genomic segments can provide insights into the evolutionary history of genes. Such information can complement phylogenies as an independent source of evidence for evolutionary relationships between paralogous (duplicated) gene lineages [25] , including MADS-box genes [26] . Therefore, we studied genomic locations of MIKC-type MADS-box genes in phylogenetically informative flowering plant genomes. To this end, we identified evolutionary conserved tandem arrangements for members of different MADS-box gene subfamilies. We observed that members of the SEP1 and SQUA , as well as SEP3 and FLC subfamilies are arranged in tandem in several core eudicot genomes ( Fig. 1 ; Supplementary Table S1 ). While members of the SQUA subfamily are exclusively next to members of the SEP1 subclade, FLC genes are consistently next to members of the SEP3 subclade. 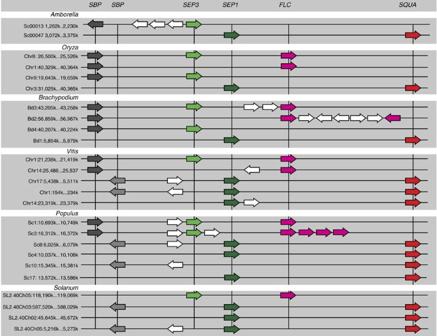Figure 1: Conserved tandem arrangements of MADS-box genes in angiosperms. Genes that exhibit conserved synteny throughout the angiosperms are represented by coloured arrows and are connected by vertical lines that are defined at the top of the figure. Loci in white did not exhibit synteny and are not discussed.SBP-like genes belonging to different monophyletic groups are differentiated by a different grey tone. On the left side of each genome fragment, position coordinates are shown. Figure 1: Conserved tandem arrangements of MADS-box genes in angiosperms. Genes that exhibit conserved synteny throughout the angiosperms are represented by coloured arrows and are connected by vertical lines that are defined at the top of the figure. Loci in white did not exhibit synteny and are not discussed. SBP -like genes belonging to different monophyletic groups are differentiated by a different grey tone. On the left side of each genome fragment, position coordinates are shown. Full size image It has been suggested that core eudicots evolved from an ancient hexaploid ancestor [27] . As such, numerous MADS-box subfamilies exhibit three core eudicot-specific subclades, for example in the SQUA and SEP1 clades [19] , [21] . In agreement with this, we observe that in Vitis , Populus and Solanum the SEP1-SQUA tandem is also present in triplicate corresponding to the different core eudicot-specific subclades ( Supplementary Table S1 ). To understand whether the genomic arrangements of MADS-box genes from the different subfamilies reflect a common evolutionary origin, we performed phylogenetic analyses including a representative sampling of subfamily members ( Fig. 2 ). We found that FLC- like genes are sister to SQUA genes in a monophyletic group that receives strong support (95 maximum-likelihood bootstrap support (BS), 1.00 Bayesian posterior probability (BPP)). Similarly, the SEP3 and SEP1 subfamilies form a monophyletic group (99 BS, 0.97 BPP), as had been observed previously [28] . SEP -like genes together with gymnosperm and angiosperm AGL6 -like genes form a supported monophyletic group (83 BS, 0.96 BBP). These gene lineages are all nested within a strongly supported superfamily, which includes SEP -, AGL6 -, SQUA - and FLC -like genes (93 BS, 0.97 BPP). Phylogenetic analysis therefore supports the idea of a common origin of these subfamilies by combination of tandem and segmental duplications. 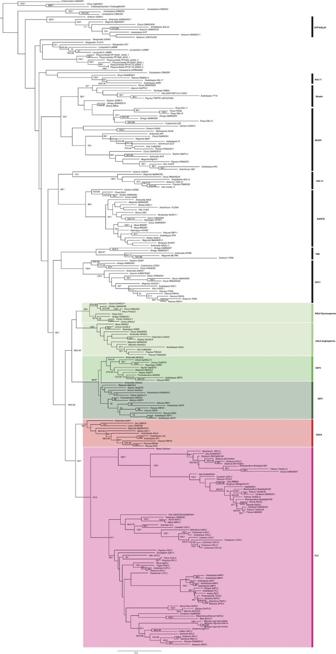Figure 2: Maximum likelihood phylogeny of MIKCc-type MADS-box genes showing the interrelationships of the different subfamilies. The numbers next to the nodes represent non-parametric BS values and Bayesian posterior probabilities for the corresponding clades. Figure 2: Maximum likelihood phylogeny of MIKC c -type MADS-box genes showing the interrelationships of the different subfamilies. The numbers next to the nodes represent non-parametric BS values and Bayesian posterior probabilities for the corresponding clades. Full size image FLOWERING LOCUS C orthologs are present in monocots SQUA and SEP1 tandem arrangements can also be identified in monocot genomes ( Fig. 1 . ). Interestingly, in monocots we identified tandems of SEP3 with MADS-box genes that are currently annotated as ‘monocot-specific’ and being related to type I or MIKC*-type MADS-box genes [29] , [30] , [31] , which are evolutionarily more ancient and structurally different lineages of MADS-box genes. The genomic position of these genes, however, suggests that they represent members of the FLC subfamily in monocots. Indeed, in the phylogeny these enigmatic monocot genes group with FLC genes from core eudicots with high BS (99 BS, 1.00 BPP, Fig. 2 ). This indicates that these genes were previously misclassified FLC orthologs in monocots. The FLC monocot clade itself is strongly supported (100 BS, 1.00 BPP) and consists solely of genes from Poaceae, except for MpFLC ( Musa paradisiaca, Musaceae). In the order Poales, we identified two major FLC clades, which we will refer to as OsMADS37 -like genes and OsMADS51 -like genes. The fact that both rice and sorghum have duplicate FLC copies could be explained by the putative whole-genome duplication 56–72 million years ago (mya) termed ‘rho’, which occurred before the divergence of the major grass lineages [25] , [32] . Subsequently, in one of these gene lineages a tandem duplication occurred, apparently before the origin of Pooideae. These monocot-specific duplications resulted in three FLC clades in temperate grasses and two major lineages in the order Poales [33] . The monocot FLC genes are characterized by divergent, short protein sequences, which probably made it difficult to identify them through traditional similarity searches, such as Basic Local Alignment Searches Tool (BLAST) [11] . In recent studies, several members of the OsMADS51 clade have been shown to function in vernalization-controlled flowering in temperate grasses similar to FLC -like genes in core-eudicots ( Supplementary Fig. S1 ) (refs 33 , 34 ). To our knowledge, no members of the OsMADS37 clade have previously been investigated. To understand the cold regulation of the different FLC paralogs in more detail, we monitored their expression level in the temperate grass model Brachypodium distachyon after 2, 4 and 6 weeks of prolonged cold (4 °C) using quantitative reverse transcription-PCR (qRT–PCR). The expression of BdMADS37 (Bradi3g41297) decreases gradually during vernalization ( Fig. 3a ). The expression of the OsMADS51 -like gene BdODDSOC2 (Bradi2g59190) is more rapidly downregulated by vernalization and a minimal expression level is reached already after 2 weeks of cold, or possibly sooner, and remained stable in subsequent weeks ( Fig. 3c ). In contrast, the expression of BdODDSOC1 (Bradi2g59120) at 4 °C mirrored the control condition during 2 and 4 weeks cold exposure, but increased after 6 weeks in vernalized plants compared with control plants ( Fig. 3b ). In conclusion, Brachypodium FLC -like paralogs are responsive to prolonged cold exposure, but the nature of the response differs both qualitatively and quantitatively between paralogs. 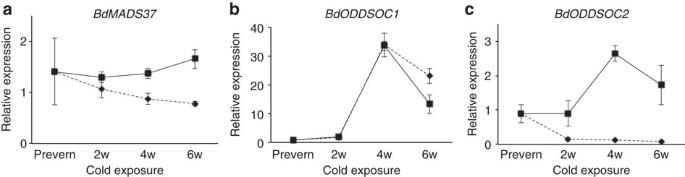Figure 3: Expression ofBrachypodium distachyon FLChomologues in response to prolonged coldBdMADS37(a),BdODDSOC1(b) andBdODDSOC2(c). Expression of FLC-like genes inBrachypodiumwere monitored using qRT–PCR in plants exposed to a 6-week-period at 4 °C (vernalized) or 28 °C (control). Expression in vernalized samples is represented by diamonds, while the control samples are indicated by squares. Prevern, prevernalization; 2w, two weeks; 4 w, four weeks; 6 w, six weeks. Error bars represent the s.e.m. of three biological replicates. Figure 3: Expression of Brachypodium distachyon FLC homologues in response to prolonged cold BdMADS37 ( a ), BdODDSOC1 ( b ) and BdODDSOC2 ( c ). Expression of FLC-like genes in Brachypodium were monitored using qRT–PCR in plants exposed to a 6-week-period at 4 °C (vernalized) or 28 °C (control). Expression in vernalized samples is represented by diamonds, while the control samples are indicated by squares. Prevern, prevernalization; 2w, two weeks; 4 w, four weeks; 6 w, six weeks. Error bars represent the s.e.m. of three biological replicates. Full size image Ancient duplication events in the MADS-box gene superclade The phylogenetic sister-relationship between the FLC / SQUA and SEP3/SEP1 clades, in combination with the SEP1-SQUA and SEP3-FLC tandem arrangements suggest a single origin of these subfamilies through ancient tandem duplication. The presence of gymnosperm AGL6 -like genes in this large superfamily of flowering time genes indicates that this tandem duplication predates the divergence of gymnosperms and angiosperms. The tandem arrangements can provide a simple explanation for the apparent absence of SEP -, SQUA - and FLC- like genes in extant gymnosperms after the split of AGL6 and SEP clades, through a single segmental deletion of the ancestral SEP - SQUA / FLC tandem along the gymnosperm stem-lineage. In agreement with the ancient evolutionary origin of the tandem arrangements, we observed that the SEP1-SQUA tandem is also present in the Amborella genome, the species sister to all other flowering plants ( Fig. 1 ). However, in Amborella neither FLC -like MADS-box genes are in tandem with SEP3 -like genes nor could we identify FLC -like genes through BLAST searches, suggesting that FLC -like genes have been lost in the lineage that led to extant Amborella . To provide additional support for the sister-relationship between FLC and SQUA and between SEP1 and SEP3 clades, we investigated the synteny of these MADS-box gene loci. We used a novel hybrid mode approach in i-ADHoRe 3.0, a program to detect large-scale synteny between genomic regions [35] . In hybrid mode, i-ADHoRe 3.0 is able to detect ancient duplication events, even in the presence of additional, more recent, whole-genome duplications. In the Vitis genome, regions around VvFLC2 were found to show significant synteny with those around VvSEP2-VvFUL and VvSEP3-VvAP1 ( Supplementary Fig. S2 ). For example, SEP3 - FLC tandems are preceded by a SQUAMOSA PROMOTER BINDING PROTEIN -like gene ( SBP ) from one monophyletic lineage, while the SEP1 - SQUA tandems are preceded by SBP genes from a monophyletic sister group ( Fig. 1 , Supplementary Fig. S3 ). These results show that the ancestral SEP and SQUA/FLC lineages underwent an apparent joint round of duplication prior to the radiation of the extant angiosperms, which resulted in the SEP1 and SEP3 clades and the SQUA and FLC clades. Based on synteny and phylogenetic relationships, these duplications were derived from the same segmental duplication in the common ancestor of angiosperms. This is consistent with the recently proposed whole-genome duplication shortly before the radiation of extant angiosperms estimated at 192±2 mya (ref. 36 ). Jiao et al . suggested that the gene duplication leading to AGL6 and SEP subfamilies was derived from a whole-genome duplication in the common ancestor of extant seed-plants [36] . If the AGL6-SEP split indeed originated from such a segmental duplication, we would expect that AGL6 is in tandem with another MADS-box gene, similar to the SEP-SQUA/FLC tandems, and that this other subfamily would be sister to the SQUA/FLC clade. While we find that AGL6 -like genes form conserved tandem arrangements with members of another MADS-box gene subfamily: the SOC1- like genes, its exact relation with the SEP - SQUA / FLC tandems will require further research ( Supplementary Note 1 ). The origin and functional diversification of developmental control genes is thought to be a major prerequisite for the evolution of complex morphological traits in eukaryotes. We elucidated the origin of three major MADS-box gene subfamilies. These subfamilies have essential roles in floral transition and flower development: the SQUA and SEP subfamilies act as positive regulators of floral transition and flower development, while FLC genes have mainly been shown to act as vernalization-responsive floral repressors in eudicots. The concept of vernalization originates from the early observation that winter varieties of cereals require prolonged cold to flower, while spring varieties flower soon after sowing [12] . Using a combined approach of synteny and phylogeny reconstruction, we were able to unambiguously identify FLC -like genes in monocots. This raises the question whether the findings for FLC in Arabidopsis can be translated to cereal crops and how FLC function diverged in flowering plants. The absence of FLC genes in monocots has previously been used as a major argument to claim an independent origin of vernalization response in these taxa [12] , [13] , [14] . In the future, it will be interesting to see to what extent functional data from Arabidopsis on FLC can be translated to its relatives in temperate cereals or vice versa and whether this can advance our understanding on the vernalization pathway in both cereals and core eudicots. Besides this, FLC genes appear to have been lost in several lineages of flowering plants ( Supplementary Fig. S4 ). It will be interesting to study the frequency and taxonomic distribution of these gene losses and how the floral transition, especially temperature response, evolved in the absence of FLC -like genes in these species. The results of functional analyses of some members of the OsMADS51 clade ( Supplementary Fig. S1 ), and also our expression data, suggest that some members of the FLC subfamily are controlled by vernalization in temperate grasses, similar to FLC in Arabidopsis. Whether this regulation by cold temperatures is conserved between eudicots and temperate grasses remains to be determined. Also the conservation of underlying gene-regulatory networks and downstream functions of FLC -like genes requires additional research. It is tempting to speculate that some aspects of FLC regulation and functions are conserved throughout angiosperms. Even more intriguingly, some members of the SQUA subfamily, which is sister to the FLC clade, are also regulated by vernalization, although in a positive manner. Examples include VERNALIZATION1 ( VRN1) in the vernalization-sensitive grass species Triticum aestivum [14] , [37] or APETALA1 and FRUITFULL in Arabidopsis thaliana whose transcript levels change in response to cold [38] . However, as also members of other MADS-box gene subfamilies, such as STMADS11 -like genes in grasses [39] , are controlled by vernalization, this type of temperature-dependent regulation may have evolved multiple times independently. The conserved SEP3-FLC and SEP1-SQUA tandem arrangements in core eudicot and monocot genomes, in combination with the phylogenetic relationships, indicate that the ancestors of these subfamilies originated from a single tandem duplication ( Fig. 4 ). The exact timing of the tandem duplication, as well as the relationship with AGL6 - SOC1 tandems, awaits additional combined synteny/phylogeny studies, including more genomes from gymnosperms, as well as basal angiosperms. It is, however, clear that before the diversification of angiosperms, a large-scale duplication, whole-genome or segmental, resulted in the duplication of the ancestral SEP - SQUA / FLC tandem, which gave rise to the SEP3 , SEP1 , SQUA and FLC gene clades in a concerted manner. 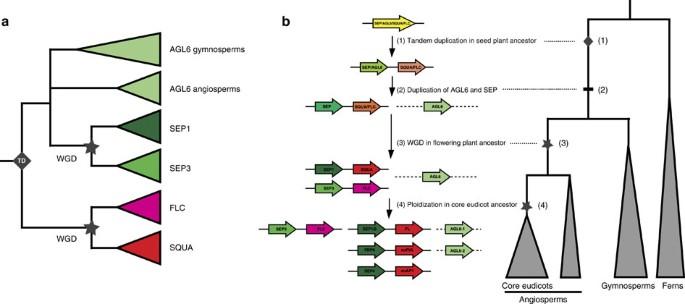Figure 4: The duplication origin ofFLC,SEPandSQUAsubfamilies. (a) Tree summarizing our current understanding of the phylogenetic relationships based on our and previous analyses. The grey diamond and grey stars denote the inferred tandem duplication (TD) and angiosperm whole-genome duplication (WGD) respectively. (b) Evolutionary scenario explaining how a single-tandem duplication and subsequent large-scale duplications expanded theSEP,AGL6,SQUAandFLClineages. Figure 4: The duplication origin of FLC , SEP and SQUA subfamilies. ( a ) Tree summarizing our current understanding of the phylogenetic relationships based on our and previous analyses. The grey diamond and grey stars denote the inferred tandem duplication (TD) and angiosperm whole-genome duplication (WGD) respectively. ( b ) Evolutionary scenario explaining how a single-tandem duplication and subsequent large-scale duplications expanded the SEP , AGL6 , SQUA and FLC lineages. Full size image Clarifying the origin and evolution of plant MADS-box gene clades is of strong interest for evolutionary developmental biologists, as it helps to trace the evolution of developmental gene-regulatory networks in plants. Bringing our findings into a larger context, the origin of major flowering MADS-box gene subfamilies by tandem duplication and subsequent segmental duplications may be linked to the elaboration of the reproductive transition process and of reproductive meristem identities. The evolutionary origin of flowering plant meristems with specific inflorescence and floral ‘identities’ is still poorly understood, and homologies of reproductive meristem identities between gymnosperms and angiosperms are debated [40] . The origin of distinct inflorescence and floral meristems may be associated with the evolution of SQUA and SEP gene functions. These genes are essential for the synorganization of reproductive meristems and primordia in the bisexual flower of angiosperms. The potential loss of these genes in gymnosperms may have had consequences for the evolution of meristem identities in these plant lineages. The investigation of gymnosperm genomes, such as the spruce genome [41] , could provide further insights into the evolution of these enigmatic genes. Local synteny Local synteny was qualitatively determined using the genome browsers implemented in Phytozome [42] , PLAZA 2.5 (ref. 43 ), the Sol Genomics Network [44] and the Amborella Genome Project ( http://www.amborella.org ; funded by the National Science Foundation grant #0922742). Tandem repeats and shared syntenic markers around SEPALLATA- and SQUAMOSA -like genes were identified by BLAST searches against the GenBank database. Detecting synteny using i-ADHoRe First, a data set was composed consisting of all angiosperm proteins from PLAZA 2.5 (ref. 43 ), combined with proteins of more recently sequenced species, Brassica rapa [45] , tomato [46] and potato [47] . Additionally the Vitis vinifera annotation was downloaded from PLAZA 2.5 and converted to input for i-ADHoRe 3.0 (ref. 35 ). An all-against-all blastp was run (version 2.2.27+ using default settings) [48] to determine pairwise similarities between all proteins in the data set. Next, using tribe-MCL [49] , the blast output was clustered into homologous gene families, with relaxed settings so even ancient homologues are included in the same gene family (settings: blast-m9, blast-ecut=1e-03, blast-score=e, mcl-I=1.2 and mcl-scheme=4). For the detection of significant synteny in grapevine, i-ADHoRe 3.0 (ref. 35 ) was used in hybrid mode, in this mode first colinear regions are detected and hidden from the data set and in a next step the remaining fraction of the genome is scanned for additional syntenic regions. (cluster_type=hybrid, cloud_gap_size=10, cloud_cluster_gap=15, cloud_filter_method=binomial_corr, gap_size=30, cluster_gap=35, q_value=0.75, alignment_method=gg2, level_2_only=false, prob_cutoff=0.001, anchor_points=3 and multiple_hypothesis_correction=FDR). A less stringent run was performed with a prob_cutoff of 0.05, cloud_gap_size=20 and cloud_cluster_gap=25. Detection of markers without synteny Vitis MADS box genes ( Supplementary Table S1 ) were extracted together with 40 protein-coding genes up- and downstream and stored as a list per gene. Redundancy due to tandems was removed and the remaining lists were screened for marker genes that could be used to provide additional insight in the origin of the SEP3-FLC , SEP1-SQUA and AGL6-SOC1 tandem arrangements. Here valid markers are sets of at least three homologous genes, which occur in proximity of all three classes MADS-box genes. Phylogenetic analyses We performed BLAST searches using core eudicot FLC sequences represented in a published FLC phylogeny [11] against the GenBank, TIGR (The Institute for Genomic Research) and AAGP (Ancestral Angiosperm Genome Project) databases to retrieve additional core eudicot FLC -like genes. Based on the observation of conserved tandem repeat arrangements in core eudicot genomes between SEP3 -, SEP1 -, SQUA- and FLC -like genes, we found OsMADS37 as a candidate FLC -like sequence in rice. This sequence was used in BLASTN searches to identify similar sequences present in the Genbank database and all sequences retrieved were included in a data matrix for phylogenetic analysis. In addition, we putatively identified the ODDSOC2 clade from the Barley ( Hordeum ) EST collection through weaker similarity with OsMADS37 . Using BLAST searches similar sequences were included in further analyses. We attempted to comprehensively sample all major subfamilies of MIKC c -type MADS-box genes [50] to investigate the evolutionary affinities of the sequences found. These subfamilies were consistently represented by sequences of at least one asterid, rosid, magnoliophyte, monocot and gymnosperm when available. Finally, known charophyte, moss and fern MIKC c -type MADS-box genes were included. Using the above sampling rationale we obtained a nucleotide data-matrix consisting of 254 sequences, which was aligned using MAFFT v6 (ref. 51 ) and manually refined using MacClade4 (ref. 52 ). The sequences used in phylogenetic analyses are listed in Supplementary Table S3 . C-terminal sequences could not be unambiguously aligned and were therefore excluded from the alignment. In addition, several gene specific insertions were also removed which resulted in a final alignment of 528 bp. The jModeltest program [53] was used to determine the best-fit model of nucleotide substitution according to the Akaike information criterion, which selected the GTR+I+G evolutionary model. The maximum-likelihood phylogenetic analysis was performed using PhyML 3.0 (ref. 54 ). Bootstrap values summarize 100 bootstrap replicates. Bayesian analysis was carried out using MrBayes 3.2 (ref. 55 ). Two independent runs with each 4 Markov Chain Monte Carlo chains were run for 15,000,000 generations and sampled every 1,000 generations. After convergence indicated by a s.d. of split frequencies <0.02, we removed the first 25% of the sampled trees as burn-in. The posterior distribution over trees is presented as a majority-rule consensus tree and posterior probabilities are indicated at their respective nodes. Both trees were rooted using charophyte MIKC c type MADS-box genes. qRT–PCR of FLC -like genes in Brachypodium Brachypodium distachyon plants were grown in pots containing 50:50 soil:vermiculite. Plantlets were pregrown under long-days (16 h light-8 h dark; 54 photons μmol m −2 s −1 ) at 28 °C until the third leaf fully emerged. These ‘three-leaf’ plantlets were subsequently transferred to another growth chamber at 4 °C (vernalization treatment) or 28 °C (control) (16 h light-8 h dark; 20 photons μmol m −2 s −1 ) during 6 weeks and plants were harvested prevernalization and at 2, 4, and 6 weeks. Immediately after harvesting, samples were flash frozen in liquid nitrogen. RNA was extracted from whole plants with their root removed using Trizol (Invitrogen, Carlsbad, USA). Subsequently all RNA samples were DNase treated using TURBO DNA-free (Ambion, Austin, USA). Complementary DNA was prepared by reverse transcription using AMV reverse transcriptase (Promega, Madison, USA). qRT–PCR was performed on a StepOne Plus apparatus (Applied Biosystems, Foster City, USA) using Fast SYBR Green Master Mix (Applied Biosystems, Foster City, USA). The ubiquitin-conjugating enzyme 18 gene ( UBC18; Bradi4g00660) was used as a reference gene to normalize the samples [56] . Relative gene expression change was calculated using the delta-delta C t method. Error bars represent the s.e. of three biological replicates, which are the mean of three technical replicates. The following primers were used for qRT–PCR: Bradi2g59187 (F: 5′-AAATCCAAGATATTGGCAAAACG-3′, R: 5′-CCTTAGGCTCACTGGAGTTCTCA-3′), Bradi2g59120 (F: 5′-CCGGCAAGCTCTACGAGTACTC-3′, R: 5′-GCTCCCGCAAATTGCTGAT-3′, Bradi3g41297 (F: 5′-CAATCTGAGGATGAAGGTGTCACA-3′, R: 5′-GCTTGACAAGTTGTTCGCTTTCT-3′) and UBC18 (F: 5′-GTCGACTTCCCCGAGCATTA-3′, R: 5′-ATAGGCGCCGGGTTGAG-3′). How to cite this article: Ruelens, P. et al. FLOWERING LOCUS C in monocots and the tandem origin of angiosperm-specific MADS-box genes. Nat. Commun. 4:2280 doi: 10.1038/ncomms3280 (2013).